Crystal structure of listeriolysin O reveals molecular details of oligomerization and pore formation Listeriolysin O (LLO) is an essential virulence factor of Listeria monocytogenes that causes listeriosis. Listeria monocytogenes owes its ability to live within cells to the pH- and temperature-dependent pore-forming activity of LLO, which is unique among cholesterol-dependent cytolysins. LLO enables the bacteria to cross the phagosomal membrane and is also involved in activation of cellular processes, including the modulation of gene expression or intracellular Ca 2+ oscillations. Neither the pore-forming mechanism nor the mechanisms triggering the signalling processes in the host cell are known in detail. Here, we report the crystal structure of LLO, in which we identified regions important for oligomerization and pore formation. Mutants were characterized by determining their haemolytic and Ca 2+ uptake activity. We analysed the pore formation of LLO and its variants on erythrocyte ghosts by electron microscopy and show that pore formation requires precise interface interactions during toxin oligomerization on the membrane. Pore-forming toxins (PFTs) that disrupt the plasma membrane of mammalian cells are the most common bacterial virulence factors. More than 25% of all cytotoxic bacterial proteins are PFTs, and they are found in virtually all important classes of pathogens [1] . Well-known examples include the hemolysins of the Gram-negative bacteria Escherichia coli , Aeromonas hydrophilia or Vibrio cholerae as well as the haemolytic PFTs produced by Gram-positive pathogens such as Staphylococcus aureus, Streptococcus pneumoniae and Listeria monocytogenes . PFTs are classified as α- or β-PFTs according to the α-helix or β-barrel structure they form after penetrating the host cell membrane. Listeriolysin O (LLO) is the crucial virulence factor produced by the Gram-positive pathogen L. monocytogenes . It is a member of the family of cholesterol-dependent cytolysins (CDC), which comprise the largest family among bacterial PFTs [2] . A sequence identity of 40–70% suggests that all members have similar tertiary structures and a conserved basic mechanism of action [3] . CDC monomers are secreted by the pathogenic bacteria in a water-soluble form that binds to a receptor on the target cell, where they oligomerize into a ring of up to 50 monomers with a diameter of around 300 Å [4] , [5] . Pore formation occurs through a subsequent conformational change, in which two helix bundles in each monomer convert into a pair of amphiphilic transmembrane β-hairpins that insert into the membrane [3] , [6] , [7] . Membrane insertion of CDCs results in characteristic features that range from changes in ion fluxes across damaged membranes to cell lysis. It has become apparent that prelytic concentrations of toxins have a multitude of effects on the host cell. It has been known for some time that low concentrations of intracellular toxin affect host cell signalling in various ways, including activation of the p38 mitogen-activated protein kinase [8] , the c-Jun N-terminal pathways [9] and induction of pattern recognition receptors such as the NALP3 inflammasome [10] . In addition, LLO has been implicated in inducing autophagy [11] as well as in the suppression of reactive oxygen species produced by the NOX2 NADPH oxidase [12] . Over the past few years it has emerged that LLO activates diverse cellular processes including the dysregulation of post-translational modifications mediated by SUMOlyation [13] , induction of endoplasmic reticulum stress and reversible fragmentation of mitochondria [14] as well as regulatory epigenetic changes due to the post-translational modification of histone tails [15] . The most heterogeneous region of CDCs is their N-terminal sequence, which harbours distinct functions for some of the family members. Streptolysin O (SLO) from Streptococcus pyogens depends on its N-terminal sequence for translocating NAD-glycohydrolase across the host cell membrane [16] . The N-terminal extension of Lectinolysin from Streptococcus mitis is a fucose-binding lectin domain (glycan binding site) modulating pore-forming activity [17] . The proline/serine-rich N-terminus of LLO resembles a eukaryotic PEST-like sequence and ensures that the phagosomal membrane but not the host plasma membrane is disrupted, as the host cytosol is the replicative niche of L. monocytogenes [18] . Mutations within this region increase the cytotoxicity of Listeria and result in a higher permeability of the host plasma membrane. This decreases the virulence of the bacteria by exposing the host cytosol, including the Listeria itself, to extracellular defenses [19] . Early models proposed a proteasomal degradation of LLO in the cytosol upon ubiquitination and phosphorylation of its N-terminus [18] . However, intracellular lifetimes of both wild-type LLO (LLO WT ) and PEST sequence mutants are similarly short, making it unlikely that proteasomal degradation regulates LLO in the host cytosol [20] . The cytoplasmic inactivation of LLO could also be the result of temperature-dependent denaturation [21] or oligomerization/aggregation of LLO [22] , respectively. Research on PFTs, in particular CDCs, is of great medical interest because of their essential function as virulence factors for pathogenic bacteria. LLO takes a special position among the CDCs as it enables L. monocytogenes to live inside host cells, a feature that is not shared by other CDC-producing bacteria [23] . In addition, LLO is a promising target for the development of antitumor vaccines [24] . Interestingly, bacterial CDCs and eukaryotic pore-forming proteins such as perforin [25] , C6, C8α and C8β have in overall very similar structures and they most likely follow a similar mode of action when spanning the membrane [26] , [27] , [28] , [29] . Here, we present the crystal structure of natively produced LLO from L. monocytogenes in its secreted, water-soluble monomeric form. We show that the N-terminal PEST-like sequence forms a left handed polyproline type II helix and delineate how this helix is involved in intra- and intermolecular interaction of LLO. We show which residues are implicated in the predicted pH sensor, and describe several hydrophilic and ionic interactions at the interface of the membrane-inserting regions of the toxin, which are likely involved in the pH- and temperature-dependent regulation of LLO. In the crystals, we found LLO monomers in a linear side-by-side arrangement and identified critical residues at the interface that are involved in row formation. Haemolysis and Ca 2+ uptake experiments demonstrated the importance of these residues for LLO activity. We show by electron microscopy (EM) that the monomer interface is important for LLO oligomerization and for pore formation in the membrane. Crystal structure of LLO Diffraction data from three-dimensional crystals of natively secreted LLO were used for structure determination by molecular replacement [30] with Perfringolysin O (PFO) [31] as a search model. Overall, the structure of LLO resembles that of the related CDCs PFO [31] , Anthrolysin O [32] , Intermedilysin [33] , Suilysin [34] and the recently published SLO [35] . LLO is an elongated, rod-like molecule with four distinct domains, referred to as D1 to D4 ( Fig. 1 ). D1 has an α/β fold with a five-stranded β-sheet and is surrounded by six α-helices. D2 has four β-strands and forms a three-stranded antiparallel β-sheet that connects D1 to D4. D3 consists of a five-stranded antiparallel β-sheet, which is surrounded by six α-helices in an α/β/α-fold. D4 is a compact β-sandwich comprising two four-stranded β-sheets. Whereas D1, D2, and D3 are intertwined, D4 appears to be an independent folding unit connected to D2 via a glycine (G417). The undecapeptide 483 ECTGLAWEWWR 493 , which is highly conserved among the CDCs, and the loops involved in receptor recognition and initial membrane binding are located on the side of D4 that faces away from D2. The signal peptide comprising amino acids 1–24 is cleaved off during secretion and therefore absent in the mature molecule. The N-terminal extension of LLO known as ‘PEST-like sequence’ interacts with the β-sheet surface of D1 ( Fig. 2 ) as well as with the adjacent, symmetry-related molecule. 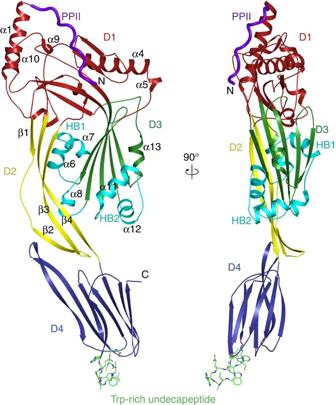Figure 1: LLO crystal structure. Cartoon representation of the LLO crystal structure. The individual domains are shown in different colours. PPII helix is shown in purple, D1 in red, D2 in yellow, D3 in green and D4 in blue. The membrane-inserting helix bundles (HB1 and HB2) in D3 are shown in cyan. The tryptophan-rich undecapeptide at the tip of D4 is presented as stick model in green. Figure 1: LLO crystal structure. Cartoon representation of the LLO crystal structure. The individual domains are shown in different colours. PPII helix is shown in purple, D1 in red, D2 in yellow, D3 in green and D4 in blue. The membrane-inserting helix bundles (HB1 and HB2) in D3 are shown in cyan. The tryptophan-rich undecapeptide at the tip of D4 is presented as stick model in green. 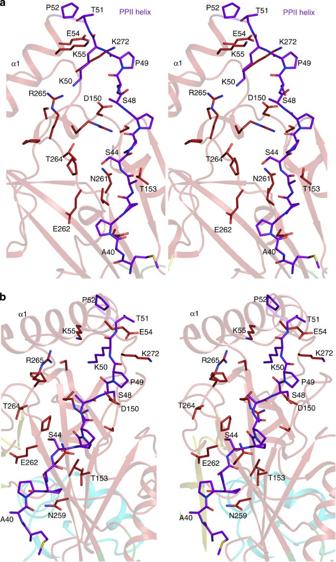Figure 2: Molecular interactions of the N-terminal PPII helix. 3D stereo views of domain D1 with the PPII helix shown in purple in stick representation seen from two different directions (a,b). Full size image Figure 2: Molecular interactions of the N-terminal PPII helix. 3D stereo views of domain D1 with the PPII helix shown in purple in stick representation seen from two different directions ( a , b ). Full size image PPII helix The PEST-like sequence makes LLO unique amongst the CDCs. This region is proposed to play a key role in protein compartmentalization and regulation that restrict the pore-forming activity to the host cell vacuole. While the PEST-like sequence (aa 39–51) is well resolved ( Fig. 2 ), the preceding residues 25–38 are, due to their flexibility, not visible in the structure. Due to the six prolines, it adopts a four-turn left-handed helix without intramolecular hydrogen bonds, owing to the proline torsion angles. This arrangement is also known as a polyproline type II (PPII) helix, a conspicuous feature found in many protein structures [36] . The PPII helix of LLO is located laterally above D1 and points towards the neighbouring, symmetry-related molecule in the crystal lattice. Further, it stabilizes the long, solvent-exposed helix α1, which in turn interacts with the loop-connecting helices α9 and α10 and is well conserved among Listeria species ( Fig. 3 ). 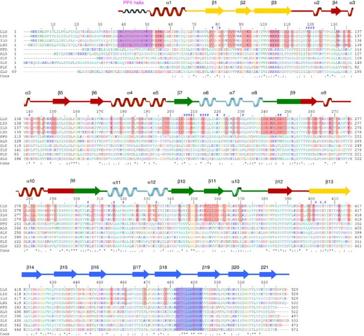Figure 3: Sequence alignment of CDCs from selected bacteria. The first four rows show LLO sequences from genusListeria. The LLO PPII helix sequence and undecapeptide are highlighted in purple and blue, respectively. The residues conserved inListeriaare highlighted in red. A ‘#’ indicates residues found in the cluster formed by the membrane-inserting helix bundles and their neighbours. Elements of secondary structure, colours and sequence numbers correspond to the LLO crystal structure shown inFig. 1. (SeeSupplementary Table 1for the accession codes of the protein sequences used.) Figure 3: Sequence alignment of CDCs from selected bacteria. The first four rows show LLO sequences from genus Listeria . The LLO PPII helix sequence and undecapeptide are highlighted in purple and blue, respectively. The residues conserved in Listeria are highlighted in red. A ‘#’ indicates residues found in the cluster formed by the membrane-inserting helix bundles and their neighbours. Elements of secondary structure, colours and sequence numbers correspond to the LLO crystal structure shown in Fig. 1 . (See Supplementary Table 1 for the accession codes of the protein sequences used.) Full size image The PPII helix contains three putative phosphorylation sites (S44, S48 and T51), of which S44 can be phosphorylated in vitro by the mammalian MAP kinase Erk2 (ref. 20) [20] . All three sites face the D1 surface but their environments are quite different. T51 in the region connecting PPII to helix α1 is exposed to the solvent and interacts weakly with E54 of helix α1. S48 is closer to domain D1 and is hydrogen-bonded to D150 in the loop connecting β5 and β6. S44 interacts most closely with D1, forming a hydrogen-bonding network with surface residues N261 and T264 ( Fig. 2 ). The residues interacting with S44 and S48 and holding PPII on the D1 surface are largely present in Listeria species but are poorly conserved among other CDCs ( Fig. 3 ). pH and temperature regulation of LLO The pore-forming activity of LLO depends on pH and temperature. On the basis of a LLO model, the three acidic residues D208, E247 and D320 in domain D3 were identified as a pH sensor [21] . The LLO crystal structure now shows that one Na + and a water molecule mediate the interactions of D208, E247 and Y206 from the central β-sheet with D320 and K316 from the second membrane-inserting helix bundle (HB2, Fig. 4a ). Furthermore, we identified five additional clusters with extensive networks of ionic and hydrophilic interactions at the boundary of the first helix bundle (HB1) with the surrounding domains D1, D2, and the central β-sheet coordinating in total 7 Na + and 18 H 2 O ( Fig. 4b–f ). The second cluster is located at the backside of the central β-sheet. Here, D207 and E209 interact via two Na + and three H 2 O with K220 and Q216 of helix α6 and with Y406 from D2 ( Fig. 4b ). The third cluster is at the interface of D1, D2 and HB1 where N140 and N402 from domain D1 and D2, respectively, and T223 from HB1 interact with the main-chain oxygen of I218 via one Na + and three H 2 O ( Fig. 4c ). In cluster four, Y348 from the central β-sheet contacts the main chain of a loop connecting β-strand β3 to helix α2 of D1 via one Na + and three H 2 O ( Fig. 4d ). Interactions between side chains and the main chain also occur in the next cluster where E246, K305 and K344 from the central β-sheet interact with the loop-connecting helices α7 and α8 ( Fig. 4e ). One Na + and three H 2 O mediate tight interactions of S213, E214 and S215 in TMH1 with Y78, D81 and S404 from D2 β-sheet to form the last cluster on the reverse of helix α6 ( Fig. 4f ). 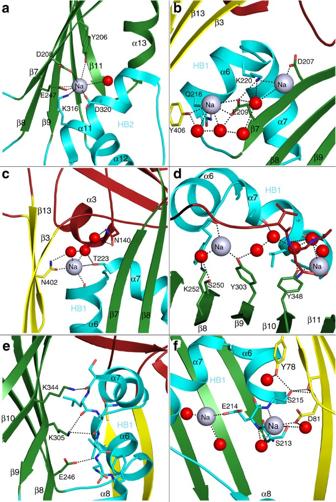Figure 4: Interaction clusters stabilizing both membrane-inserting helix bundles in the ‘locked’ conformation. Na+ions and H2O are shown as grey and red spheres, respectively. (a) The initially as ‘acidic triad’ predicted cluster is formed by D208/E247/Y206 from the central β-sheet and K316/D320 from α11 of the second membrane-inserting helix bundle. (b) Y406 from domain D2 β-sheet interacts in the second cluster with the acidic residues D207/E209 of the central β-sheet and Q216/K220 of α6. (c) The next cluster forms the interface of D1, D2 with α6 and α7 via the coordination of one Na+and three H2O through N140, N402 and T223. (d) S250/K252 from β8, Y303 from β9, and Y348 from β10, interact with α6 and D1 via two Na+and six H2O. (e) Side chains of E246, K306 and K344 from the central β-sheet interact with the main chain of the loop connecting α7 to α8. (f) S213/215 and E214 from α8 and Y78/D81/S404 from D2 β-sheet make tight hydrophilic and ionic interactions to form the last cluster. Figure 4: Interaction clusters stabilizing both membrane-inserting helix bundles in the ‘locked’ conformation. Na + ions and H 2 O are shown as grey and red spheres, respectively. ( a ) The initially as ‘acidic triad’ predicted cluster is formed by D208/E247/Y206 from the central β-sheet and K316/D320 from α11 of the second membrane-inserting helix bundle. ( b ) Y406 from domain D2 β-sheet interacts in the second cluster with the acidic residues D207/E209 of the central β-sheet and Q216/K220 of α6. ( c ) The next cluster forms the interface of D1, D2 with α6 and α7 via the coordination of one Na + and three H 2 O through N140, N402 and T223. ( d ) S250/K252 from β8, Y303 from β9, and Y348 from β10, interact with α6 and D1 via two Na + and six H 2 O. ( e ) Side chains of E246, K306 and K344 from the central β-sheet interact with the main chain of the loop connecting α7 to α8. ( f ) S213/215 and E214 from α8 and Y78/D81/S404 from D2 β-sheet make tight hydrophilic and ionic interactions to form the last cluster. Full size image We calculated the pKa of all ionizable residues in the interface of HB1/2 in the presence and absence of Na + ions and found that the residues on both sides of the central β-sheet, including Y206, D208 and E247 of the pH sensor, show conspicuous pKa shifts as compared with the free state ( Supplementary Table 2 ). A sequence alignment ( Fig. 3 ) in combination with structural mapping ( Fig. 5 ) shows residues conserved in Listeria , which may regulate the pH and temperature dependence of LLO. We found an accumulation of such residues on both sides of the central β-sheet (240–248). These residues are sandwiched between HB1/2 and the tip of β2 (91–94), which is surrounded by HB2 and domain D4 where K93 forms a salt bridge to D416. In addition to the pH-sensitive clusters described above, changes in pH and temperature would also affect the salt bridge K93/D416 and hence affect the relative orientation of D4 at the point where it connects to D2 via its glycine linker (G417). 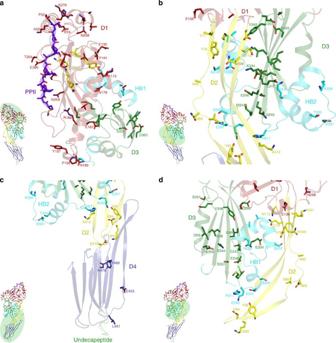Figure 5:Residues conserved inListeria. Location of amino acids conserved in LLO from differentListeriaspecies shown as stick model. The overall location is highlighted in green on the small overall structure. (a) PPII helix and domain D1 residues. (b) Residues of the central β-sheet, membrane-inserting helix bundle 2 (HB2) of D3 and domain D2. (c) Domain D4 and the interface of D4, D2 and D3. (d) Domain D2, the back of the central β-sheet and membrane-inserting helix bundle 1 (HB1). Figure 5: Residues conserved in Listeria. Location of amino acids conserved in LLO from different Listeria species shown as stick model. The overall location is highlighted in green on the small overall structure. ( a ) PPII helix and domain D1 residues. ( b ) Residues of the central β-sheet, membrane-inserting helix bundle 2 (HB2) of D3 and domain D2. ( c ) Domain D4 and the interface of D4, D2 and D3. ( d ) Domain D2, the back of the central β-sheet and membrane-inserting helix bundle 1 (HB1). Full size image Residues involved in oligomer formation In the LLO crystals, individual molecules form linear arrays along the short unit cell axis ( Fig. 6a,c ). The striking charge complementarity in domains D1 and D3 of adjacent molecules ( Fig. 6d ) suggests that these regions might be important for intermolecular contacts, and therefore for oligomer and pore formation. To test this hypothesis, we introduced mutations in this region ( Fig. 7a ), determined their haemolytic activity on sheep erythrocytes and compared them with LLO WT ( Fig. 7c,d ). Deletion of the PPII helix (LLO ΔPPII ) or mutations within this helix (LLO A40W , LLO S44D , LLO S44E ) increased the haemolytic activity of LLO. We also observed a significant increase in activity for the D1 mutant LLO D394W . In contrast, the mutations of K175 to glutamate (LLO K175E ) or E262 to lysine (LLO E262K ), which invert the charge on the interface, render LLO virtually inactive. The replacement of S176 by a voluminous tryptophan (LLO S176W ) likewise abolished haemolytic activity, while the replacement of E262 by tryptophan (LLO E262W ) did not show any influence on the haemolytic activity. On the other hand, the D3 mutation LLO N230W reduced the haemolytic activity to around 50% of LLO WT . These results show clearly that the interface between adjacent LLO molecules in the crystal structure is functionally important and mutations have a major effect on oligomer formation and haemolytic activity. Circular dichroism (CD) spectra of inactive mutants and WT are similar, suggesting that all have the same secondary structure and are correctly folded ( Fig. 7b ). 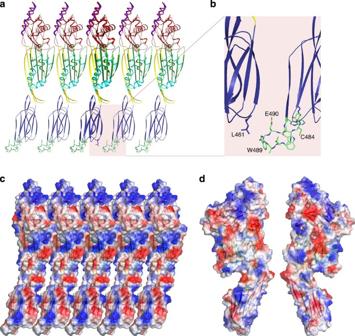Figure 6: Intermolecular interface of the crystal rows. (a) Cartoon representation of LLO monomers forming a linear array. (b) Detailed view of the intermolecular interactions of L461 with the undecapeptide of the neighbouring molecule. L461 and the undecapeptide are shown as ball-and-sticks in A and B. (c) Surface potential representation of LLO monomers forming a linear array. (d) Charge complementary of the surface forming the interface between two monomers. Figure 6: Intermolecular interface of the crystal rows. ( a ) Cartoon representation of LLO monomers forming a linear array. ( b ) Detailed view of the intermolecular interactions of L461 with the undecapeptide of the neighbouring molecule. L461 and the undecapeptide are shown as ball-and-sticks in A and B. ( c ) Surface potential representation of LLO monomers forming a linear array. ( d ) Charge complementary of the surface forming the interface between two monomers. 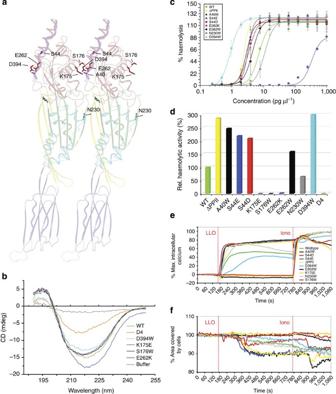Figure 7: Activity measurements of LLO interface mutants. (a) Location of the mutated residues in the interface of two monomers. (b) CD spectrum of selected LLO mutants. (c) Haemolytic activity of the selected LLO mutants. The activity, determined by three measurements is shown as a function of the toxin concentration and the error bars represent s.d. The non-haemolytic mutants LLOK175E, LLOS176Wand LLO D4 were not included in the graph. (d) Comparison of the haemolytic activity relative to the wild type. (e) Calcium uptake activity of selected mutants. The activity is expressed relative to Ca2+uptake facilitated after application of ionomycin. Mean values of three independent experiments are shown. (f) Cell surface shrinking of epithelial monolayers upon LLO incubation and Ca2+influx. Full size image Figure 7: Activity measurements of LLO interface mutants. ( a ) Location of the mutated residues in the interface of two monomers. ( b ) CD spectrum of selected LLO mutants. ( c ) Haemolytic activity of the selected LLO mutants. The activity, determined by three measurements is shown as a function of the toxin concentration and the error bars represent s.d. The non-haemolytic mutants LLO K175E , LLO S176W and LLO D4 were not included in the graph. ( d ) Comparison of the haemolytic activity relative to the wild type. ( e ) Calcium uptake activity of selected mutants. The activity is expressed relative to Ca 2+ uptake facilitated after application of ionomycin. Mean values of three independent experiments are shown. ( f ) Cell surface shrinking of epithelial monolayers upon LLO incubation and Ca 2+ influx. Full size image Ca 2+ uptake At sublytic concentrations, LLO facilitates the influx of Ca 2+ from the extracellular medium into the cell or causes the release of Ca 2+ from intracellular stores into the cytosol [37] . In either case, increased levels of cytosolic free Ca 2+ disturb cellular Ca 2+ homeostasis, which results in release of proinflammatory mediators, changes in cellular metabolism, reorganization of the cytoskeleton and ultimately apoptosis [38] , [39] . Other deleterious effects of increased Ca 2+ levels observed at early stages of Listeria infection include loss of cell volume, change of cell size and a weakening of the epithelial monolayer [40] . We therefore hypothesized that LLO forms Ca 2+ channels in the plasma membrane. To characterize Ca 2+ uptake of LLO mutants ( Fig. 7a ), we determined their ability to form Ca 2+ channels in Caco-2 epithelial cells by monitoring intracellular Ca 2+ levels and cell volume on incubation with 50 ng ml −1 LLO or variants ( Fig. 7e,f ). Consistent with the haemolytic activity ( Fig. 7c,d ), the PPII mutations in LLO A40W , LLO S44D , LLO S44E and the PPII helix deletion in LLO ΔPPII clearly increased Ca 2+ influx and cell shrinkage, while no influx or cell shrinkage was observed for the mutants with completely abolished haemolytic activity (LLO K175E , LLO S176W ). Also LLO E262W was not able to facilitate Ca 2+ influx, whereas it showed slightly increased haemolytic activity. While the haemolytic activity of LLO N230W was slightly lower, Ca 2+ uptake was initially higher, resembling that of LLO WT after 10 min. By contrast, Ca 2+ uptake of LLO D394W was at first lower but almost reached WT levels eventually. Oligomer formation of LLO on erythrocyte membranes The molecular details of the mechanisms by which CDCs oligomerize and form the membrane-inserting pore are still unknown. The crystal structure of LLO shows linear interactions between protomers that would be expected in the initial oligomer after membrane binding. The structure therefore serves as a model for studying the intermolecular interactions that result in pore formation. So far we have shown how changes of interface residues affect haemolytic activity and Ca 2+ uptake. However, a reduced activity might also result from a hindered oligomerization or inhibited transition from the initial oligomer to a prepore or pore. To investigate this further, we examined the structures of LLO WT and mutants on the membrane of erythrocyte ghosts by transmission EM. LLO WT mostly forms complete rings of variable size on ghost membranes ( Fig. 8 ). Incomplete rings and arcs were also found occasionally next to the ghosts, which we assume have become detached from the membrane. As expected, all LLO mutants that were haemolytic or facilitated Ca 2+ uptake (LLO ΔPPII , LLO A40W , LLO S44D , LLO S44E , LLO N230W , LLO E262W ) also formed rings on the membranes. By contrast, the non-haemolytic mutants did not form rings or pores ( Fig. 8h,i,k , Supplementary Fig. 1 ). The ability of the haemolytic mutants to assemble into pores differs widely. Compared with LLO WT , the pores and rings of the PPII mutants (LLO ΔPPII , LLO A40W , LLO S44D , and LLO S44E ) with increased Ca 2+ uptake and haemolytic activity look quite different ( Fig. 8d–g ). Apart from the pore-forming full circles on the membrane surface there are many more incomplete and less curved arcs, often arranged in crowded rows on shredded ghosts. Although the interface mutant with reduced haemolytic activity (LLO N230W ) is still able to form rings, the number of complete rings visible on the ghost membranes was considerably reduced ( Fig. 8j ), whereas the rings of LLO E262W were very similar to LLO WT ( Fig. 8l ), consistent with its slightly increased haemolytic activity. The non-haemolytic LLO mutants LLO K175E , LLO S176W and LLO E262K produced discontinuous protein fibres or exhibited granulated protein structures that covered the membrane surface. No ring-like structures were found on or around the membranes, and the ghosts appeared apparently intact. The curvature of arched structures visible on the ghosts was clearly different from that of the rings and pores formed by LLO WT . Evidently, while these mutants were still able to bind to ghost membranes and to oligomerize, they did not form the characteristic lytic rings observed with LLO WT . 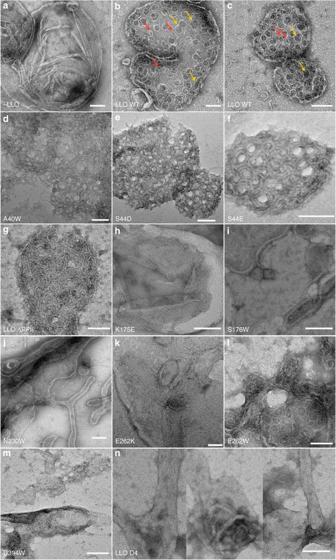Figure 8: Oligomerization of LLO mutants on erythrocyte ghosts. Erythrocyte ghosts incubated with equal amounts of LLO protein were negatively stained and imaged with a transmission electron microscope at acceleration voltage of 120 kV. (a) Erythrocyte ghosts in the absence of LLO. (b,c) Ghosts incubated with LLOWT. Red arrows point to slit-like pores and yellow arrows point to pores, which probably arose by fusion of rings. (d–m) Ghosts incubated with the indicated LLO variants. (n) Ghosts incubated with LLO domain D4 forming linear and curved oligomers. SeeSupplementary Fig. 1for more detailed views of K175E, S176W, E262K, andSupplementary Fig. 2for LLO D4. Scale bar, 100 nm. Figure 8: Oligomerization of LLO mutants on erythrocyte ghosts. Erythrocyte ghosts incubated with equal amounts of LLO protein were negatively stained and imaged with a transmission electron microscope at acceleration voltage of 120 kV. ( a ) Erythrocyte ghosts in the absence of LLO. ( b , c ) Ghosts incubated with LLO WT . Red arrows point to slit-like pores and yellow arrows point to pores, which probably arose by fusion of rings. ( d – m ) Ghosts incubated with the indicated LLO variants. ( n ) Ghosts incubated with LLO domain D4 forming linear and curved oligomers. See Supplementary Fig. 1 for more detailed views of K175E, S176W, E262K, and Supplementary Fig. 2 for LLO D4. Scale bar, 100 nm. Full size image Role of domain D4 in oligomer formation and pH inactivation Domain D4 of the CDCs plays an important role in cholesterol recognition and facilitates the initial binding to cholesterol-containing target membranes. In contrast to the intertwined domains D1–D3, domain D4 is a separate folding unit with a compact β-sandwich structure. Refolded D4 of SLO and pyolysin (PLO) have been found to bind to membranes [41] and to form linear arrays on cholesterol crystals [42] . To examine whether D4 binds to and oligomerizes on the membrane in a similar way, we expressed and purified LLO domain D4 and incubated ghosts with the purified protein. LLO D4 likewise formed long linear arrays on ghost membranes ( Fig. 8n , Supplementary Fig. 2 ). Surprisingly, the LLO D4 domain also formed curved oligomers similar to those observed for the non-lytic LLO mutants LLO K175E and LLO S176W ( Fig. 8 , Supplementary Fig. 1 ). The curvature resembles that found for LLO WT , but there are no circular structures, indicating that D4 does not assemble into complete rings. In contrast to the lytic LLO variants, incubation with D4 did not result in perforated or fragmented ghosts, consistent with our observation that LLO D4 does not lyse cells ( Fig. 7d ). Mixing of LLO D4 in ratios of 1:1, 2:1 and 3:1 (D4:WT) did not change the haemolytic activity of LLO WT ( Supplementary Fig. 3 ), whereas SLO D4 inhibited and PLO D4 amplified the activity of SLO [41] and PLO [43] , respectively. An interesting site within LLO D4 is L461 between β16 and β17. In non-listerial CDCs, the leucine at this position is replaced by a threonine. Mutation of this leucine to threonine protects LLO against pH inactivation by stabilizing the protein at higher pH and temperature [21] . In the LLO oligomer rows observed in the crystals, the distance of L461 and W489 in the conserved undecapeptide 483 ECTGLAWEWWR 493 on the surface of the neighbouring molecule is less than 4 Å ( Fig. 6b ). It has been postulated that the primary function of LLO is the release of L . monocytogenes from the phagosomal vacuole into the host cytosol. Therefore, LLO activity should be restricted to the acidic environment of the phagosome. It has previously been reported that LLO activity is regulated via a pH sensor consisting of the three acidic residues E247, D208 and D320 (the ‘acidic triad’) [21] . Deprotonation of these acidic residues at the higher pH of the cytosol would result in charge repulsion, which in turn would trigger the inactivation of LLO by unfolding and aggregation of HB1 and HB2 in domain D3. In the structure of LLO, these three residues indeed interact with each other, both directly and via bound Na + and H 2 O. We find that a tyrosine (Y206) and a lysine (K316) also contribute to this pH-sensitive cluster. The LLO crystal structure shows also an extended cluster of side-chain interactions on the boundary of HB1, similar to the cluster between HB2 and central β-sheet. The calculated pKa of ionizable residues, especially in the clusters, differ from that of amino acids in their free state and depend on the presence of ions (Na + ). Among residues showing a high pKa variance, we found the functionally important residues of the pH sensor and residues of the second acidic cluster at the interface of HB1 ( Supplementary Table 2 ). The earlier finding that high salt concentration (500 mM NaCl) prevents denaturation or aggregation at pH 7 and 37 °C [21] is fully consistent with our observation that LLO precipitates when the salt concentration drops below 50 mM (ref. 30 ). Evidently, Na + ions compensate for the negative charge of deprotonated carboxyl side chains in the cluster and thus help to keep HB1/2 folded. This suggests a complex interaction network regulating the phagosomal activity and cytoplasmic inactivation of LLO. Thus, the molecular regulation of pH dependence seems to be much more complex than initially thought and might depend to the ion concentration of the surrounding medium [21] . To demonstrate that the monomer interface seen in the crystal structure is in fact important for oligomer formation, we introduced mutations into regions of close contact or charge complementarity. Three of the selected mutations either abolished haemolytic activity (LLO K175E and LLO S176W ) or reduced it significantly (LLO E262K ). This suggests that the crystal structure does indeed show the interactions essential for the oligomerization and pore formation in atomic detail. The loss of activity in these mutants may have several possible reasons: (1) the mutations prevent membrane binding, (2) oligomer formation on the membrane is inhibited so that the mutant LLOs cannot form arcs or ring-shaped structures like LLO WT or (3) the membrane insertion of the HB1/2 is inhibited. Transmission EM of erythrocyte ghost membranes incubated with mutant LLOs clearly shows that the main reason for the loss of activity is the inability of the mutants to oligomerize into ring-shaped pores. The non-haemolytic mutants LLO K175E , LLO S176W , and LLO E262K formed irregular rows and granular protein structures on the membrane surface, similar to domain D4 alone, indicating that they were still able to bind the membrane but unable to form complete rings with a curvature that appears to be necessary for pore formation and lysis. The sporadically observed ring and arc formation for LLO N230W shows that this mutation is obviously not able to prevent the monomer interactions. The mutation of D394 to tryptophan in LLO D394W also did not prevent ring formation on erythrocyte ghosts. The haemolytic activity of this mutant was even significantly higher, whereas Ca 2+ uptake was lower. This may be due to a higher salt sensitivity of this mutant. At the lower salt concentrations used for the Ca 2+ uptake experiments and CD spectroscopy ( Fig. 7b ), a fraction of the protein precipitated. This would reduce the effective protein concentration, which would explain the lower Ca 2+ uptake activity. A L. monocytogenes recombinant strain expressing a LLO K175A variant exhibited reduced plaque-forming ability (44% that of WT) [44] , indicating that it is still able to form pores in the phagosome. In contrast, the mutant LLO K175E described here completely lacks activity and would probably not be able to allow Listeria to escape from the phagosome, thus resembling a ΔLLO mutant [45] . This suggests that an alanine in place of K175 does not prevent the formation of oligomers or pores, as was the case with K175E. The observed reduction in haemolytic activity of K175A can therefore be ascribed to a loss of charge complementarity due to the missing counter-charge for E262. Also the charge inverting mutation of E262 to lysine, but not to tryptophan, renders LLO inactive, indicating that the match of charges at this position is more critical than the match of the surface. It has previously been shown that SLO D4 is able to bind to membranes and inhibit the haemolytic activity of full-length SLO [41] . PLO D4 also is able to bind to membranes [43] and to form straight arrays on cholesterol crystals [42] . In contrast to SLO D4, addition of PLO D4 to the full-length protein amplifies its haemolytic activity, whereas added LLO D4 does not, indicating that this domain probably does not integrate into the oligomers. We also show that LLO D4 forms linear or curved arrays on ghost membranes, suggesting that D4 does more than promoting the initial binding of LLO to the membrane, it contributes to the intermolecular interactions during oligomer formation on the membrane similar to D1. The interactions of LLO D4 in the oligomers are presumably also mediated by the loops that contain the conserved undecapeptide and L461, which in non-listerial CDC is a threonine. In LLO, a threonine at this position shifted the equilibrium towards oligomerization, resulting in increased activity at higher pH and temperature [21] . LLO mutations that eliminate the haemolytic activity of LLO also eliminate the LLO-mediated Ca 2+ influx and cell shrinkage at sublytic toxin concentrations. This suggests that charge and surface complementarity are equally important for the haemolytic activity of LLO and for the formation of Ca 2+ channels. We demonstrate that (1) the Ca 2+ channels are formed by LLO rather than by another molecule, (2) channel and pore formation are closely linked and (3) both are the result of LLO oligomerization. The LLO oligomer of the Ca 2+ channels must be different from that of the large haemolytic pore. At present, it is unknown how many LLO monomers combine to form such channels, and how they interact. Previous patch clamp studies proposed at least three LLO monomers for the formation of a functional pore [37] . We propose that LLO monomers associate on the membrane by surface charge complementarity followed by membrane insertion of their β-hairpins to form a narrow β-barrel channel. At high toxin concentrations, we often observe that LLO WT pores on the ghost membranes differ in size and shape. Occasionally, in addition to full-circled pores we also see rings, arcs, incomplete rings and slit-shaped structures ( Fig. 8b,c ), which may arise from the fusion of arcs or rings. This correlates reasonably with the ‘growing pore’ model [46] where the toxin binds and immediately inserts the membrane to form small pores, which successively grow to full-size pores. Whether LLO also forms complete prepore rings, as in the case of pneumolysin [7] and PFO [47] remains to be shown experimentally, for example, by locking LLO in a prepore form like PFO [47] . However, at sublytic toxin concentrations (<500 ng ml −1 ), we see no structures on the ghosts in our EM analysis that could be correlated with Ca 2+ influx. As the toxin concentrations used for the EM analysis were certainly much higher, we can only speculate whether such slit-like structures are also present at the sublytic concentrations used for the Ca 2+ influx measurement. It is possible that similar structures are responsible for the Ca 2+ influx and loss of cell volume at sublytic LLO concentrations. It has been proposed that the PPII helix is involved in LLO inactivation by proteolysis in the host cytosol and that removal of this helix leads to loss of virulence by dysregulated lysis of the host cell plasma membrane [18] . However, the half-lives of wild-type and PPII mutants are similar and both are stabilized by proteasome inhibitors, making proteasome degradation unlikely [20] . An alternative role for the PPII helix has been postulated in transcriptional control, whereby LLO translation is negatively regulated during the logarithmic growth phase by control elements within the PPII sequence of the LLO mRNA [48] . Silent mutations within this mRNA region result in increased levels of LLO in the cytosol, rendering these mutants less virulent. Our data indicate a regulatory role in pore formation for the PPII helix region at protein level. The PPII helix between the LLO molecules in the linear arrays including its flexible N-terminal region would interfere with the formation of an optimal curvature and therefore reduce the ring formation, resulting in downregulation of LLO activity. Accordingly, one possible mechanism for the inactivation of LLO in the host cytosol would be the interaction of the PPII helix with host cell cytosolic proteins, which might fix the helix to the interaction surface, thus inhibiting or preventing LLO oligomerization and pore formation. These interactions of LLO with cytosolic proteins could induce the cellular responses observed in the presence of LLO. One of the consequences of the prevented ring formation would be the inactivation by unfolding of HB1/2 and subsequent aggregation or degradation. Deletion of PPII helix or mutations that support the displacement of the PPII helix from the D1 surface would thus aid the formation of ring-shaped oligomers ( Fig. 9 ) and pores. This is borne out by our haemolysis experiments showing that the corresponding mutants are indeed more active than wild type. We conclude that subunit interactions across the protomer interface are essential for LLO oligomerization and slight variations here have high impact on the ability of LLO to form ring-shaped oligomers. 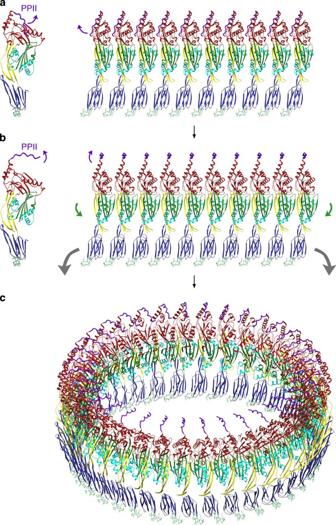Figure 9: Model of LLO oligomerization, ring formation and the role of the PPII helix. (a) In the model, insertion of the N-terminal PPII helix between monomers prevents the formation of oligomers with optimal curvature for membrane insertion. Interaction with cytosolic proteins may affect the location of the PPII helix at the D1 surface. (b) Displacement of the PPII helix (purple arrow) aids the formation of an optimally curved oligomer (green arrows) and subsequent pore formation (grey arrows). (c) Model of one ring composed of 36 LLO monomers rotated by 10° relative to the neighbouring molecule and translated by one unit cell. Figure 9: Model of LLO oligomerization, ring formation and the role of the PPII helix. ( a ) In the model, insertion of the N-terminal PPII helix between monomers prevents the formation of oligomers with optimal curvature for membrane insertion. Interaction with cytosolic proteins may affect the location of the PPII helix at the D1 surface. ( b ) Displacement of the PPII helix (purple arrow) aids the formation of an optimally curved oligomer (green arrows) and subsequent pore formation (grey arrows). ( c ) Model of one ring composed of 36 LLO monomers rotated by 10° relative to the neighbouring molecule and translated by one unit cell. Full size image Site-directed mutagenesis Site-directed mutagenesis was performed with the QuikChange site-directed mutagenesis kit (Stratagene) according to the manufacturer’s instructions with the wild-type construct as a template and primers listed in Supplementary Table 3 . All constructs were verified by nucleotide sequencing. Protein expression and purification For 3D crystallization, natively produced LLO WT was secreted into the expression medium and purified in one step by ion exchange chromatography [49] . For biochemical investigation, the LLO proteins (LLO WT and mutants) without secretion signal (amino acids 1–24) were heterologously produced in E. coli BL21 (DE3). For expression with an N-terminal His 6 -tag, gene segments encoding residues 25–529 of LLO WT , various LLO mutants or the 51–529 construct (LLO ΔPPII ) were cloned into the plasmid pET15b. Domain D4 (residues 415–529) was cloned into pGEX6p1 for N-terminal GST fusion. An overnight preculture was transferred to ‘terrific broth’ medium containing 100 μg ml −1 ampicillin. On reaching an A 600 of 1.2 at 37 °C, protein expression was induced with 1 mM isopropyl β- D -1-thiogalactopyranoside, and the temperature was lowered to 30 °C. After 4 h, cells were pelleted, resuspended in lysis buffer (50 mM Tris pH 7.7, 150 mM NaCl) and disrupted with a Microfluidizer (M-110L, Microfluidics Corp., Newton, MA). After 1 h of centrifugation at 12,000 g , the cell-free supernatant containing the His 6 -tagged constructs was loaded onto a Ni-NTA column. The protein was eluted by cleaving the His 6 -tag with thrombin on the Ni-NTA column. Eluted protein was concentrated (30 kDa cutoff) and loaded onto a gel filtration column (Superdex200) with 25 mM Tris (pH 7.7), 150 mM NaCl as running buffer. For purification of GST-tagged D4, the cell-free supernatant was loaded onto a GSH4B column, and eluted with running buffer containing 20 mM reduced glutathione. After cleavage of the fusion protein with Prescission protease, a gel filtration run (Superdex75) was carried out to separate domain D4 from GST. Fractions containing LLO were concentrated to 5 mg ml −1 , snap-frozen in liquid nitrogen and stored at −80 °C. CD spectroscopy CD spectra were acquired on a Jasco J-810 spectrometer at 298 K with a 0.2 mm cuvette at a protein concentration of 0.5 mg ml −1 in 25 mM Tris–HCl, pH 7.0, 150 mM NaCl. The spectra were recorded every 0.5 nm in the wavelength range of 190–250 nm and visualized with the Origin data analysis software package. Structure determination, refinement and structure analysis Natively produced [49] LLO WT has been crystallized [30] by the hanging-drop vapour diffusion technique and data were collected at 100 K on European Synchrotron Radiation Facility microfocus beam-line ID23-2. Data processing, integration and scaling were performed with the XDS package [50] . The structure was solved by molecular replacement with PFO (pdb-id 1PFO) as the search model using PHASER [51] from the CCP4 software package [52] . The initial electron density map covering only the search model was extended automatically by cycles of density modification, automatic model building using RESOLVE [53] and refinement by REFMAC5 (ref. 54) [54] . The model was subjected to iterative rounds of rebuilding into 2F o −F c and F o −F c electron density maps using COOT [55] and refined using the phenix.refine subroutine from the PHENIX programme suite [56] . Data collection, refinement and model statistics are summarized in Table 1 . Figures were generated with Pymol [57] . Salt-dependent pKa values were calculated using pdb2pqr [58] . Table 1 Data collection and refinement statistics. Full size table Haemolysis assay The haemolytic activity of LLO was determined by lysis of sheep erythrocytes [49] . Purified protein was serially diluted in haemolysis buffer (50 mM sodium phosphate pH 6.6, 150 mM NaCl, 5 mM dithiothreitol (DTT), 0.1% (v/v) bovine serum albumin) in final volumes of 50 μl and incubated for 30 min. at 37 °C with 50 μl of a suspension of erythrocytes (I0 8 ml −1 ). The released haemoglobin was determined by measuring the optical absorbance at 405 nm. The amount of toxin necessary to lyse 50% of erythrocytes was determined and expressed as percentage of the value for LLO WT . The absorbance upon incubation with 1% Triton-X-100 or adding of 50 μl H 2 O was used as reference value for 100% lysis of the erythrocytes. Three independent measurements were performed for each LLO mutant. Specimen preparation and EM Standard haemoglobin-free unsealed ghosts were prepared [59] , diluted (1:20) in resealing buffer (11 mM Tris–HCl pH 7.6, 130 mM KCl, 10 mM NaCl, 3 mM MgCl 2 ) and incubated for 30 min. at 37 °C. The resealed ghosts were spun down for 20 min. at 12.000 g and transferred into the reaction buffer (150 mM NaCl, 50 mM sodium phosphate pH 6.6, 5 mM DTT). After the addition of LLO at 5 μg ml −1 , the mixture was incubated for 30 min at 37 °C. LLO-treated erythrocytes were transferred to EM grids and stained with 1% (wt/vol) uranyl acetate. Negatively stained specimens were analysed with an FEI Tecnai Spirit transmission electron microscope operating at an acceleration voltage of 120 kV. Images were recorded on a Gatan 2K × 2K CCD camera at a magnification of 25,000 × –45,000 × and 1.0–1.5 μm defocus. Ca 2+ -influx and cell surface measurements Caco-2 cells were loaded with 5 μM Fura-2 AM, incubated for 40 min at 37 °C and 5% CO 2 and then placed in microscopy chambers with 1 ml of HEPES medium (1.2 mM KH 2 PO 4 , 2.6 mM KCl, 2.25 mM MgSO 4 , 1.2 mM NaCl, 25 mM HEPES pH 7.4, 2.5 mM glucose, 1.3 mM CaCl 2 ). For activation LLO was preincubated with 5 mM DTT for 10 min at room temperature and added at 50 ng ml −1 to the cells. A video imaging system for fluorescence microscopy was used to measure the changes in intracellular calcium concentrations. The experimental setup allowed the simultaneous recording of the total surface area covered by cells. Changes in intracellular calcium [Ca 2+ ] i concentrations were recorded by the software as changes in the ratio of 340/380 nm. Three independent measurements were performed for each LLO mutant. The data collected from these experiments were shown as percentage of the maximum possible signal induced by adding 5 μM of the ionophore Ionomycin 10 min after LLO treatment. Accession codes: Coordinates and structure factors have been deposited at the Protein Data Bank with the accession code 4CDB . How to cite this article: Köster, S. et al. Crystal structure of listeriolysin O reveals molecular details of oligomerization and pore formation. Nat. Commun. 5:3690 doi: 10.1038/ncomms4690 (2014).